High genome heterozygosity and endemic genetic recombination in the wheat stripe rust fungus Stripe rust, caused by Puccinia striiformis f. sp. tritici ( Pst ), is one of the most destructive diseases of wheat. Here we report a 110-Mb draft sequence of Pst isolate CY32, obtained using a ‘fosmid-to-fosmid’ strategy, to better understand its race evolution and pathogenesis. The Pst genome is highly heterozygous and contains 25,288 protein-coding genes. Compared with non-obligate fungal pathogens, Pst has a more diverse gene composition and more genes encoding secreted proteins. Re-sequencing analysis indicates significant genetic variation among six isolates collected from different continents. Approximately 35% of SNPs are in the coding sequence regions, and half of them are non-synonymous. High genetic diversity in Pst suggests that sexual reproduction has an important role in the origin of different regional races. Our results show the effectiveness of the ‘fosmid-to-fosmid’ strategy for sequencing dikaryotic genomes and the feasibility of genome analysis to understand race evolution in Pst and other obligate pathogens. Stem, leaf and stripe rust diseases of wheat caused by Puccinia graminis f. sp. tritici ( Pgt ), P. triticina ( Pt ) and P. striiformis f. sp. tritici ( Pst ) have caused significant yield losses during epidemics that have resulted in famines throughout human history. They continue to threaten worldwide wheat production and global food security [1] , [2] , [3] . To prevent wheat rust epidemics, an international consortium known as the Borlaug Global Rust Initiative ( http://www.globalrust.org/ ) was established. Of the three wheat rust diseases, stripe rust occurs most frequently in the United States, primarily due to infection during the early growing season, long-distance air-borne spore dispersal and a recent adaptation to warmer temperatures [4] , [5] . Although Pst populations in most areas around the world have low genetic diversity due to clonal asexual reproduction, high levels of genetic diversity have been observed in some Pst populations from western China and central Asia [6] , [7] . Recently, Berberis species were reported to serve as the alternate host of Pst in western China and United States [8] , [9] . Therefore, sexual reproduction may be an important factor accounting for genetic variation in Pst , and regions in central Asia may serve as the centres of origin for new races. Better understanding of virulence variations and mechanisms of rust fungus–wheat interactions is necessary for the development and deployment of more effective and durable resistant cultivars [10] . However, wheat rust fungi are obligate biotrophic pathogens that cannot be cultured on artificial media. Most of their life stages, including urediniospores that are commonly used for aetiological and evolutionary biology studies, are dikaryotic ( Fig. 1 ). Therefore, it is extremely difficult to conduct molecular studies and functional characterizations of genes in rust fungi [10] , [11] . Nevertheless, recent technological advances have enabled the use of genomic approaches to study virulence variation, development and evolution in rust and other obligate biotrophic fungi [12] , [13] . 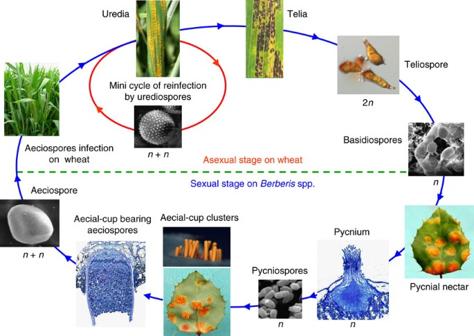Figure 1: Life cycle ofPuccinia striiformisWestend f. sp.tritici. In most of the wheat-growing regions worldwide, urediniopores are the only inoculum for the initial and recurrent infection of wheat plants, which is known as the mini cycle ofPst. Although the alternate host was identified recently, the role of sexual reproduction in genetic variation and race evolution ofPstis largely unknown. Figure 1: Life cycle of Puccinia striiformis Westend f. sp. tritici . In most of the wheat-growing regions worldwide, urediniopores are the only inoculum for the initial and recurrent infection of wheat plants, which is known as the mini cycle of Pst . Although the alternate host was identified recently, the role of sexual reproduction in genetic variation and race evolution of Pst is largely unknown. Full size image Among the rust fungi that have been sequenced, the genome sequences of Pgt and Melampsora larici-populina ( Mlp ) were generated by Sanger sequencing [12] . In 2011, a rough draft sequence of a US isolate of Pst was generated with short reads from next-generation sequencing (NGS) [14] . All of these rust genome projects used genomic DNA isolated from dikaryotic (N+N) urediniospores for sequencing analyses. The two nuclei in urediniospores are highly heterozygous in rust fungi, a characteristic that has confounded genome assembly by conventional approaches, especially with short NGS reads. The coverage and contig integrity of the released Pst draft sequence (contig N50 of 5 kb) were obviously hampered by the heterozygosity [14] . In this study, we generate a significantly improved draft genome (~110 Mb) of a Chinese Pst isolate, CY32, using a ‘fosmid-to-fosmid’ sequencing strategy that combines the use of a fosmid library and Illumina sequencing. This isolate has been the most prevalent virulent strain in China since 1991 and caused severe yield losses in the 2002 wheat stripe rust epidemic [15] . The assembled genome sequence of CY32 is 130.7 Mb, which is approximately twice as large as the released Pst- 130 genome (64.8 Mb) [14] . Our results show that the ‘fosmid-to-fosmid’ strategy is more effective than the conventional whole-genome shotgun (WGS) approach for sequencing dikaryotic rust fungi. In addition, we resequence five prevalent Pst isolates collected from different geographical locations. We identify a large number of SNPs using whole-genome comparative analyses between Pst -CY32 and individual re-sequenced isolates. Approximately 35% of SNPs are in the coding sequence (CDS) regions and half of them are non-synonymous, indicating significant genetic variation among these Pst isolates. Our re-sequencing data implies a significant role for sexual reproduction in evolution of Pst races. Genome sequencing and assembly A genomic DNA library consisting of 19,200 fosmid clones with an average insert size of 36 kb was constructed (~6.3-fold genome coverage) and randomly pooled into 1,920 pools (10 clones per pool). Each of the barcoded pools (each with a unique index) was sequenced to ~228-fold depth using Illumina GA and assembled separately using SOAP de novo [16] , [17] (‘fosmid-to-fosmid’). The primary assembled contigs were used for simulating sequencing and merged into large fragmental reafs (supercontigs) with the overlap layout consensus (OLC) [18] to generate the secondary assembly. Self-to-self whole-genome alignment with LASTZ and sequencing depth information were used to remove redundancy in the assembly [19] . The WGS sequencing approach was employed to sequence paired-ends (PE) genomic libraries that had an average insert size of 200 bp to 6 kb with Illumina GA. The resulting Illumina PE reads (average of 67 bp) in combination with mate pair information from fosmid-pooling reads were used for scaffolding of all the reafs (supercontigs) after filtering out low-quality reads. Because urediniospores used for DNA isolation were harvested from infected wheat leaves instead of sterile cultures, the assembled scaffolds were searched against the nucleotide database to remove possible contamination from plant, bacteria and insects ( Supplementary Fig. S1 ). The combined length of assembled scaffolds is 130.7 Mb. The N50 of scaffolds and contigs reach 125 kb and 18 kb, respectively, which is a significant improvement compared with the Pst draft assembled solely with WGS Illumina reads ( Table 1 ). Table 1 Features of the Pst -CY32 dikaryotic genome draft. Full size table The Pst genome size was estimated with Illumina sequencing data of three WGS PE libraries (with average insert sizes of 224, 311 and 515 bp, respectively) based on k-mer (k-base fragment) analysis [20] and the distribution of contig length and depth. Two peaks (16 and 30) were identified in the 17 k-mer depth distribution of WGS Illumina reads ( Fig. 2a ), and similarly, two peaks of coverage (Cvg) (7 and 17) were identified in the distribution of contig length and depth ( Fig. 2b ), indicating that the two haploid nuclei of Pst urediniospores differ significantly in genome sequences. Considering the heterozygous nature of dikaryotic urediniospores, the haploid genome size of Pst was estimated to be ~110 Mb ( Supplementary Fig. S2 , Supplementary Tables S1–S4 , Supplementary Notes 1 and 2 ). 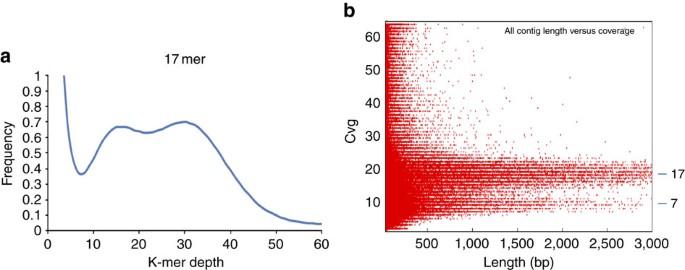Figure 2: The K-mer distribution and contig frequency analysis. (a) Seventeen k-mer depth distribution of whole-genome Illumina reads. Two peaks at 16 and 30 were identified. (b) Two peaks of Cvg 7 and 17 were identified in the distribution of contig length and depth. These results indicated that the two haploid nuclei ofPsturediniospore are highly heterozygous. The haploid genome size can be estimated using a modified Lander–Waterman algorithm based on K-mer analysis (Supplementary Notes 1 and 2). K-mer, a unique sequence ofknucleotides long; Cvg, coverage. Figure 2: The K-mer distribution and contig frequency analysis. ( a ) Seventeen k-mer depth distribution of whole-genome Illumina reads. Two peaks at 16 and 30 were identified. ( b ) Two peaks of Cvg 7 and 17 were identified in the distribution of contig length and depth. These results indicated that the two haploid nuclei of Pst urediniospore are highly heterozygous. The haploid genome size can be estimated using a modified Lander–Waterman algorithm based on K-mer analysis ( Supplementary Notes 1 and 2 ). K-mer, a unique sequence of k nucleotides long; Cvg, coverage. Full size image Approximately 49% of the Pst genome assembly consists of transposable elements (TEs) or repetitive sequences. The class I LTR retro-elements and class II terminal inverted repeat (TIR) DNA transposons are among the most abundant ones and account for ~27% and ~17% of the Pst genome, respectively. The same pipeline was used to identify the TE or repetitive sequences in the other two sequenced rust fungi, Pgt and Mlp . We found that the proportion of TEs or repeats in the Pgt and Mlp genomes was ~48% and ~49%, respectively ( Supplementary Tables S5–S7 ). Whereas the Mlp genome is enriched for TIR class II DNA transposons and DIRS class I retrotransposons, the Pgt genome has more LTR class I retrotransposons ( Supplementary Fig. S3 ). The role of these TEs in the evolution of rust genomes requires further investigation. Validation of sequence assembly To validate the ‘fosmid-to-fosmid’ assembly of the Pst -CY32 genome, 10 randomly selected fosmids were individually sequenced from end to end by Sanger sequencing. The mapped ratio of assembled scaffolds of Illumina reads to the Sanger-sequenced fosmids reached 98.53% ( Supplementary Table S8 ). Nine of them were well covered by assembled scaffolds of Pst -CY32. The other Sanger-sequenced fosmid contained highly repetitive sequences or SV (structural variation) regions, which was revealed by alignment with unfiltered contigs and Illumina paired-end sequences ( Supplementary Fig. S4 ). In comparison with the Pst -130 assembly solely using WGS Illumina sequences, the ‘fosmid-to-fosmid’ strategy significantly improved the assembly integrity of the highly heterozygous Pst genome. For example, scaffold 475 of Pst -CY32 contains only one PE sequence-supported gap in the region that matched fosmid_txjkx and 11 contigs of the Pst -130 assembly ( Fig. 3 ). The same phenomenon was observed in other Sanger-sequenced fosmids. On average, the ratio of Pst -130 contigs to matching Pst -CY32 scaffolds is 7.2 ( Supplementary Fig. S4 ). 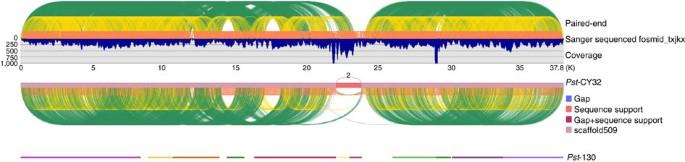Figure 3: Evaluation of assembly integrity. Scaffold 475 of thePst-CY32 assembly has only one PE supported gap, and it matches to one region of fosmid clone_Txjkx that was fully sequenced by Sanger sequencing. The same region consists of 11 contigs in thePst-130 assembly generated solely by WGS Illumina sequencing. Therefore, the fosmid-to-fosmid strategy greatly improved assembly integrity. High PE (paired end) support density indicates high assembly confidence. PE supported gaps are regions that may have SVs derived from genome heterozygosity. Green, yellow and orange curves show paired-end supports from sequences of 6-, 2- and <1-kb insert libraries, respectively. Figure 3: Evaluation of assembly integrity. Scaffold 475 of the Pst -CY32 assembly has only one PE supported gap, and it matches to one region of fosmid clone_Txjkx that was fully sequenced by Sanger sequencing. The same region consists of 11 contigs in the Pst -130 assembly generated solely by WGS Illumina sequencing. Therefore, the fosmid-to-fosmid strategy greatly improved assembly integrity. High PE (paired end) support density indicates high assembly confidence. PE supported gaps are regions that may have SVs derived from genome heterozygosity. Green, yellow and orange curves show paired-end supports from sequences of 6-, 2- and <1-kb insert libraries, respectively. Full size image A total of 1,861 expressed sequence tags (ESTs) from CY32 complementary DNA libraries constructed with RNA isolated from urediniospores, germ tubes and haustoria also were used to validate the assembly coverage. For ESTs longer than 500 bp, the coverage by the genome assembly reached 98.92% ( Supplementary Table S9 ). Reciprocal blasting analysis of Pst- coding sequences against those of Pgt and Mlp revealed that over 70% of the predicted Pst genes (17,901 genes) have support in the other two rust genomes ( Fig. 4 ). These results reflect a relatively high confidence for the assembly. 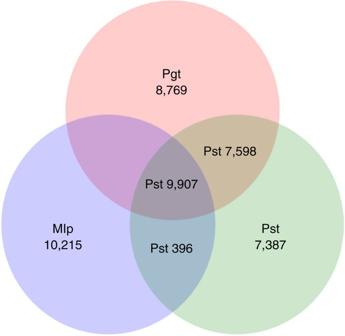Figure 4: Reciprocal Blast analysis ofPstcoding sequences againstPgtandMlp. Venn diagram showing reciprocal Blast search results for orthologous coding sequences ofPst,PgtandMlp(e-value of 1e−7). For genes with multiple alternative transcripts, the transcript with the best alignment was selected. Figure 4: Reciprocal Blast analysis of Pst coding sequences against Pgt and Mlp . Venn diagram showing reciprocal Blast search results for orthologous coding sequences of Pst , Pgt and Mlp ( e -value of 1e −7 ). For genes with multiple alternative transcripts, the transcript with the best alignment was selected. Full size image Analysis of the ultra-conserved core eukaryotic genes (CEGs) by CEGMA [21] indicates that the Pst -CY32 genome assembly has 215 complete and 7 partial models of 248 CEGs (~94%), indicating a high degree of completeness of the genome draft ( Supplementary Table S10 ). Comparative analysis with the Pst -130 genome sequence In comparison with the Pst -130 genome (64.8 Mb) assembled solely with WGS Illumina reads [14] , the Pst -CY32 genome generated by the ‘fosmid-to-fosmid’ method increased the N50 value from 5 kb to 18 kb for contigs and from 5 kb to 125 kb for scaffolds. The estimated genome size of Pst was increased to 110 Mb. More than 5.3 Mb of scaffolds that contain 1,519 predicted genes of Pst -CY32 were absent in the published Pst -130 genome ( e -value 1e −10 ). Heterozygous features in the genome of dikaryotic Pst High coverage and deep reads (26 × ) allowed the identification of 83,736 heterozygous single-nucleotide variants (SNVs) within the sequenced Pst -CY32 genome ( Supplementary Data 1 ). The heterozygosity rate (0.68 × 10 −3 ) was ~1.6 times higher than that of human (0.43 × 10 −3 ) [22] , [23] . Therefore, the two nuclei in urediniospores of Pst- CY32 must be highly heterozygous. In comparison with the estimated genome size, the current assembly is significantly larger and possesses more than 20-Mb assembly ‘redundancy’. Systematic analyses of sequences of highly similar scaffolds revealed that a set of 1,059 genes was present in the overlapping regions of scaffolds with different kinds of overlapping relationships ( Supplementary Data 2 ). The heterozygous regions and distinctive SNV genotypes of the two nuclei of Pst -CY32 were revealed by aligning sequences of assembly scaffolds with matching Sanger-sequenced fosmids. Some of the predicted genes were located in the heterozygous regions of the dikaryotic Pst genome, implying that these ‘redundancy’ genes may result from heterozygous features in the dikaryotic Pst genome ( Fig. 5 ). The ‘fosmid-to-fosmid’ strategy allowed us to independently sequence and assemble heterozygous regions that were represented in different fosmid pools, which is an advantage for investigating highly heterozygous genomic regions of dikaryotic rust fungi. 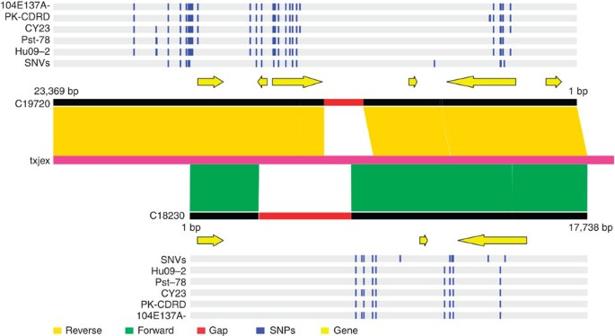Figure 5: Heterozygous regions in thePstgenome. Heterozygous regions were identified by aligning the sequence of Txjex, a fosmid fully sequenced by Sanger sequencing with c19720 and c18230, two highly similar scaffolds of thePst-CY32 assembly generated with Illumina sequences from fosmid pools 7PB_Index52_Index26/20PB_Index47_Index8 and 14PB_Index44_Index29_Index6_Index35, respectively. SNPs between the referencePst-CY32 genome and re-sequenced strains Hu09-2,Pst-78, CY23, PK-CDRD or 104E137A- are marked with blue vertical lines. SNV, heterozygous SNV in the dikaryoticPst-CY32 genome. Figure 5: Heterozygous regions in the Pst genome. Heterozygous regions were identified by aligning the sequence of Txjex, a fosmid fully sequenced by Sanger sequencing with c19720 and c18230, two highly similar scaffolds of the Pst -CY32 assembly generated with Illumina sequences from fosmid pools 7PB_Index52_Index26/20PB_Index47_Index8 and 14PB_Index44_Index29_Index6_Index35, respectively. SNPs between the reference Pst -CY32 genome and re-sequenced strains Hu09-2, Pst -78, CY23, PK-CDRD or 104E137A- are marked with blue vertical lines. SNV, heterozygous SNV in the dikaryotic Pst -CY32 genome. Full size image Annotation and comparison of three rust fungal genomes By combining automated gene calling and EST-based prediction, a total of 25,288 genes were predicted to encode peptides >50 amino acids. Whereas 1,059 of them are likely ‘redundancy genes’ related to the heterozygous nature and assembly method ( Supplementary Data 2 ), 403 genes are truncated genes ( Supplementary Data 3 ). The coding region, including introns, accounts for 33.59% of the Pst genome assembly ( Table 1 ). To assess the quality of gene prediction, we compared the length distribution of genes, CDS, exons and introns, and the distribution of exon number per Pst gene with those of related plant pathogenic fungi, including two other rust and common corn smut [12] , [24] . Pst was found to be similar to other rust fungi in all of the major parameters analysed ( Supplementary Fig. S5 ). Among all of the predicted Pst genes, only 8,334 (32.96%), 2,067 (8.17%) and 2,018 (7.98%) of them had homologues with known functions in the GO, PAMGO, and PHI databases, respectively ( Supplementary Figs S6–S8 ). Among the genes belonging to different PAMGO categories in three rust fungi, the two wheat rust fungi contained more genes involved in DNA recombination, but the gene contents in other categories were similar to those in Mlp ( Fig. 6a ). We used Hcluster_sg [25] to identify orthologues among three rust fungi. A total of 5,560 orthologous clusters were identified in two wheat rust fungi, but only 3,937 clusters were common to Pst and Mlp . The numbers of species-specific gene clusters were 4,469, 5,827 and 4,922 for Pst , Pgt and Mlp , respectively ( Fig. 6b ). These results are consistent with the closer relationship of Pgt and Pst than to Mlp . Among the genes unique to Pst in comparison with Pgt and Mlp , only 14.43% (1,066 genes) and 3.38% (250 genes) of them have homologues with known functions in the GO and PAMGO databases, reflecting inadequate investigation of gene functions in rust pathogens. Interestingly, most of known homologues belong to metabolic pathways and transport in both databases. When they were categorized into transporters, secreted proteins (SPs), kinases and carbohydrate-active enzymes (CAZY), the proportion of SP genes is higher than the others ( Fig. 6c ), consistent with observations in Mlp and Pgt [12] and suggesting the importance of SPs in virulence of rust pathogens. This phenomenon also was observed in other obligate plant pathogenic fungi, such as the powdery mildew fungus [13] . 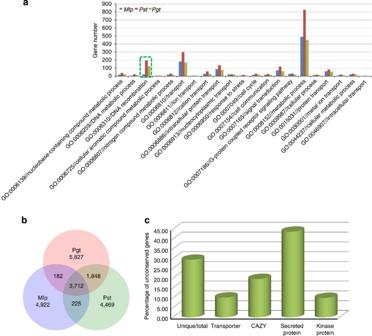Figure 6: Functional categories and comparative analysis of predictedPstgenes. (a) Functional categories and distribution of predictedPstgenes based on the PAMGO database. Among the 2,067Pstgenes categorized with the PAMGO database, major groups with 5 genes or more are presented. The most abundant functional groups belong to metabolic process, transport and DNA recombination. (b) Venn diagram showing orthologous gene clusters among thePst,PgtandMlpgenomes. For genes with multiple alternative transcripts, the transcript with the best alignment was selected. Orthologous gene families were merged into multiple species orthologous groups by MultiParanoid. (c) The result showed the percentage ofPst-specific genes in the total number of genes belonging to each gene category. Figure 6: Functional categories and comparative analysis of predicted Pst genes. ( a ) Functional categories and distribution of predicted Pst genes based on the PAMGO database. Among the 2,067 Pst genes categorized with the PAMGO database, major groups with 5 genes or more are presented. The most abundant functional groups belong to metabolic process, transport and DNA recombination. ( b ) Venn diagram showing orthologous gene clusters among the Pst , Pgt and Mlp genomes. For genes with multiple alternative transcripts, the transcript with the best alignment was selected. Orthologous gene families were merged into multiple species orthologous groups by MultiParanoid. ( c ) The result showed the percentage of Pst -specific genes in the total number of genes belonging to each gene category. Full size image Secretome A total of 2,092 proteins encoded by the Pst genome were predicted by SignalP, TargetP and TMHMM [26] , [27] , [28] , which accounts for 8.3% of the total number of proteins, and were grouped into 916 families. Similarly, the genomes of Pgt and Mlp are predicted to encode 1,459 and 1,178 SPs, respectively, accounting for 8.2% and 7.1% of the total number of Pgt and Mlp proteins. Among the putative SPs of three rust pathogens, Pst shared 341 families with the other two rust pathogens, and more than 62% of the predicted SP families were lineage-specific for Pst ( Supplementary Fig. S9 ). Furthermore, over 92% of them had no distinct orthologues in non-rust fungi, including Ustilago maydis, Blumeria graminis, Magnaporthe oryzae and Fusarium graminearum [13] , [24] , [29] , [30] . In cluster analyses, only a few predicted SPs could be grouped into small families, suggesting a substantial diversity of the Pst secretome and the lack of sequence similarity or conservation in fungal avirulence or effector genes ( Supplementary Fig. S10 ). A total of 491 SPs were distributed in 100 putative physical clusters of 2–18 members ( Supplementary Data 4 ). Twenty-seven putative SPs in Pst are homologous to seven haustorially expressed SPs (HESPs) of M. lini [31] , including Hesp-897, Hesp-735, Hesp-379, Hesp-379-like and Hesp-C49. Eighteen SPs in Pst are homologous to the rust transferred protein 1 (RTP1) [32] in other rust pathogens ( Supplementary Data 5 ). A search for known candidate effector motifs indicated that 1,052 of the Pst SP genes had the ‘Y/F/WxC’ motif of the powdery mildew fungus [33] and 114 of them had the RXLR motif reported in oomycete effectors [34] ( Supplementary Data 6 ). However, these two motifs occurred at a similar frequency in non-SPs (11,267 and 3,742 of them with the ‘Y/F/WxC’ and `RXLR' motifs, respectively). Therefore, whether Pst effectors use these sequence elements for entry into plant cells is questionable. The genomes of the obligate biotroph B. graminis , facultative biotroph U. maydis , necrotrophic pathogen F. graminearum and symbiont Laccaria bicolor [35] were found to have 442, 426, 1,049, and 1,161 SP genes, respectively, by the same scanning methodology. They account for 7.5%, 6.2%, 7.6% and 5.2% of total protein-coding genes in B. graminis , U. maydis , F. graminearum and L. bicolor , respectively. Therefore, Pst and Pgt appear to have a relatively larger secretome (higher percentage) compared with that of other plant-associated fungi. Several putative Pst effector genes were found to be specifically expressed during sexual reproduction ( Fig. 7 , Supplementary Data 7 and 8 ), suggesting that rust fungi with alternate hosts may transmit some specific SPs to cope with infection of the primary and alternate host plants. In comparison with B. graminis , U. maydis and L. bicolor , several subcategories of cell wall-hydrolyzing enzyme (CWHE) genes, particularly pectin esterase and mannanase genes, appeared to be expanded in Pst and Pgt ( Supplementary Table S11 ). Previous studies have shown that the cellulose-degrading capacity is similar among pathogens, but the ability to cope with soft tissue components, for example, hemicellulose and pectin, may vary [36] , which is consistent with our observation that expanded CWHEs in rust secretomes are mainly hemicellulases and pectinesterases. Interestingly, cutinase genes also were expanded in Pst . Although they may not be involved in wheat infection (germ tubes of Pst urediniospores invade wheat through stomata), cutinases may have an important role in Berberis infection because germ tubes produced by basidiospores directly penetrate epidermal cells of Berberis leaves [37] . 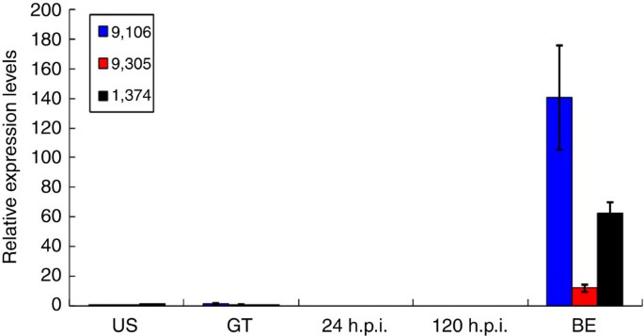Figure 7: Assays for three putativePstSP genes specifically upregulated during infection ofBerberisleaves. Pstgenes striiformis_9106, 9305, and 1374 are putative SP genes that are specifically upregulated at the pycnial stage in the infectedBerberisleaves. RNA samples were isolated from urediniospores (US), germ tubes (GT), infected wheat leaves at 24 h post inoculation (h.p.i.) or 120 h.p.i. and infected berberis (Berberis shensianaAhrendt) leaves (BE) at 11 days post inoculation (11 d.p.i.), respectively. The relative expression levels were calculated by the comparative Ct method with the elongation factor-1 gene ofPstas the internal standard. Means and s.e. were calculated from three replicates. Error bars represent the s.d. of the mean. Figure 7: Assays for three putative Pst SP genes specifically upregulated during infection of Berberis leaves. Pst genes striiformis_9106, 9305, and 1374 are putative SP genes that are specifically upregulated at the pycnial stage in the infected Berberis leaves. RNA samples were isolated from urediniospores (US), germ tubes (GT), infected wheat leaves at 24 h post inoculation (h.p.i.) or 120 h.p.i. and infected berberis ( Berberis shensiana Ahrendt) leaves (BE) at 11 days post inoculation (11 d.p.i. ), respectively. The relative expression levels were calculated by the comparative Ct method with the elongation factor-1 gene of Pst as the internal standard. Means and s.e. were calculated from three replicates. Error bars represent the s.d. of the mean. Full size image Transporters A total of 512 transporter genes, including 7 sugar and 12 amino acid transporter genes, were present in the Pst genome. Four of seven Pst genes encoding putative nucleotide sugar transporters were confirmed by qRT–PCR analysis to be highly expressed in planta . In contrast, two hexose transporters that are closely related to U. fabae HXT1 were constitutively expressed in urediniospores, germ tubes and other infection structures ( Supplementary Data 7 and 8 ), which contrasts with the expression profiles of hexose transporter genes in U. fabae [38] and M. larici-populina [12] . The Pst genome also lacks a distinct orthologue of the U. maydis srt1 sucrose transporter gene, which is similar to observations in Pgt and Mlp [12] , [39] . Thus, the rust fungi may convert sucrose to hexose by secreted invertase, and haustoria then take up hexose from host cells as the major carbohydrate source [38] , [40] . Another notable adaptation was observed in the amino acid–polyamine–organocation superfamily. Whereas the yeast genome contains only nine amino acid transporter genes, the Pst genome contains 15, indicating an expansion of the amino acid transporter family that may be related to the defect of Pst in nitrogen metabolism. Noticeably, the lack of a nitrite reductase gene in Pst will make it incapable of nitrate assimilation, which is consistent with observations in Pgt and Mlp [12] . Therefore, the uptake of amino acids from host cells by haustoria is essential for protein synthesis in Pst . Data from qRT–PCR analysis confirmed that 8 of 12 predicted amino acid transporter genes are highly expressed during Pst infection of wheat or Berberis plants ( Supplementary Data 7 and 8 ). Six of them are highly similar to PIG27 of U. fabae , which is specific for lysine and histidine [41] . Two others share homology with AAT3p and PIG2 of U. fabae [42] , [43] . Their upregulated expression in infected plant tissues supported the hypothesis that amino acid transporters are responsible for the uptake of amino acids from plant cells by haustoria [37] . Re-sequencing of five additional Pst isolates To explore the intra-specific race evolution, five additional Pst isolates from different geographical locations were selected for re-sequencing analysis ( Supplementary Table S12 ). Based on their virulence on 17 differential wheat cultivars ( Fig. 8a ), Pst -CY32 appeared to be more closely related to Pst -130 (ref. 44 ) than to CY23 and other Pst isolates. Their genomes were re-sequenced at 22-29X by the WGS strategy to a genome coverage of over 95% ( Supplementary Table S13 ). In comparison with Pst -CY32, more than 100,000 SNPs were identified in the five re-sequenced Pst isolates and 81,000 in Pst -130 (ref. 14 ). The number of SNPs is similar for individual isolates, and heterozygous SNPs occupied more than 80% of SNPs in the genomes of all six of these Pst isolates, which may be related to their heterozygous dikaryotic genomes ( Table 2 ). Based on re-sequencing data, rich SNP distribution in the heterozygous regions of Pst -CY32 could be observed, and genotypes of these five isolates are distinctive in these regions, further indicating the heterozygous property of the Pst genome ( Fig. 5 ). The number of SNPs in gene-coding regions (cSNPs) accounts for ~35% of total SNPs. Among them, half were non-synonymous mutations that may impact virulence, race specificity and other biological traits and may be responsible for adaptation to host and environmental changes. 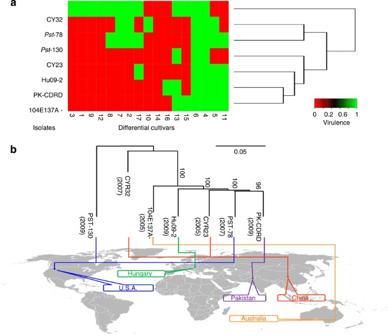Figure 8: Relationship among sevenPuccinia striiformisf. sp.triticiisolates. (a) Heat map and race relationship of 7Pstisolates according to their virulence on 17 differential cultivars. The susceptible and resistant types were recorded as 1 and 0, respectively. Heatmap.2 was used for clustering. (b) Phylogenic tree of 7Pstisolates constructed with their cSNPs using Mega5-nj. The origin and isolation date of each isolate were marked. Figure 8: Relationship among seven Puccinia striiformis f. sp. tritici isolates. ( a ) Heat map and race relationship of 7 Pst isolates according to their virulence on 17 differential cultivars. The susceptible and resistant types were recorded as 1 and 0, respectively. Heatmap.2 was used for clustering. ( b ) Phylogenic tree of 7 Pst isolates constructed with their cSNPs using Mega5-nj. The origin and isolation date of each isolate were marked. Full size image Table 2 Number and type of SNPs in five re-sequenced Pst isolates and Pst -130. Full size table Phylogenetic trees of these Pst isolates were constructed based on total SNPs and cSNPs. The topological features of the cSNP and SNP trees are similar. The Pst isolates collected from different locations exhibited significant genetic variation based on genome-wide cSNPs and could be classified into different branches ( Fig. 8b ). These results indicate that similar races may possess unexpected levels of genetic variation at the genome level. However, the SNP- or sequence-based phylogenetic tree differed from the virulence-based tree. Therefore, the evolutionary relations of Pst isolates based on SNPs were not correlated with their virulence features. For example, isolate PK-CDRD is more similar to 104E137A- in virulence than it is to Pst -78 in genome variation. Furthermore, these intra-species isolates cannot be grouped in the phylogenetic tree based on their geographical origins. Isolate Pst -78, a prevalent race in the United States, shared most recent ancestors with isolate PK-CDRD from Pakistan. Isolate Pst -130 from North America was more closely related to the Chinese isolate CY32 than to other Pst isolates. These results indicate that sexual reproduction and genetic recombination may be more important than expected for the origin of these globally dispersed isolates. We also investigated the distribution of InDels and SVs among five re-sequenced Pst isolates ( Supplementary Tables S14 and S15 ). In general, all of them are rich in InDels (1,863 on average) and SVs (759 on average), although they vary in the abundance. These results further indicate that significant genetic variation exists among these Pst isolates. Interestingly, isolate CY23, a relatively old Chinese race with a limited host range, has almost twice as many InDels as other Pst isolates in comparison with Pst -CY32 and contains only deletion-type SVs, suggesting that CY23 may differ from other Pst isolates in variations associated with race evolution and virulence. When 12 candidate Pst effector genes were selected for sequencing analysis, one of them, Gene_5778, was found to contain a 3-bp deletion in the CDS region (deletion of AGT at 346–348) in isolate CY23. The stripe rust fungus is one of the most important pathogens of wheat in the world. Although haploid basidiospores were recently found to infect Berberis species [8] , [9] , Pst exists in the dikaryotic phase during all stages of wheat infection ( Fig. 1 ). Unlike diploid organisms that contain pairs of homologous chromosomes, two nuclei in dikaryotic urediniospores formed by plasmogamy between two compatible haploid strains may be distantly related and highly heterozygous because the resulting diploids may be sterile or of low fertility. In comparison with the human genome, the Pst -CY32 genome is indeed more heterozygous. The dikaryotic nature of Pst made it extremely difficult for genome assembly, particularly with short WGS reads generated by NGS techniques. Among three rust genomes that have been published, the contig N50 for the Pst -130 assembly was only 5 kb (ref. 14 ). For the Pgt and Mlp genomes, improved assembly was achieved with longer reads from Sanger sequencing, which is much more expensive than NGS. However, over 90 Mb of the Sanger reads could not be assembled into the released 88.6-Mb Pgt genome ( http://www.broadinstitute.org ), likely due to genome heterozygosity. The current de novo genome assembly of Pst -CY32 has scaffold N50 of 125 kb, which is significantly improved over the assembly based solely on WGS sequencing. In comparison with non-rust fungal pathogens, Pst, Pgt and Mlp all have larger and more complex secretomes. Some of the expanded families of secreted proteins in Pst or other rust fungi may have important roles in fungal–plant interactions. For example, one cutinase family expanded in three rust fungi has 18, 9, and 8 members in Pst, Pgt and Mlp , respectively ( Supplementary Fig. S11 ). These cutinase genes may be important for the infection of leaves of the woody alternate host plant. Among the Pst -specific genes with homologues of known functions, the most abundant category, with over 250 members, is related to DNA replication and repair, which is consistent with the report in Pgt and Mlp [12] . Some of these genes may be related to evolutionary adaptation to environmental stresses, such as strong UV light during airborne dispersal. During the last century, spontaneous mutations were assumed to be the major source of genetic variation responsible for the emergence of new virulent races [3] , [45] . Because the alternate host was not known until 2010 (ref. 8 ), studies of the role of sexual reproduction in genetic variation and race evolution have been neglected in Pst . The re-sequencing data generated here show that similar Pst races or isolates from different continents possessed an unexpectedly large amount of genetic variation at the genome level based on SNP and InDel analyses. The phylogenetic relationship among these Pst isolates is not related to their virulence features on differential cultivars or to their geographical origins. All these data from comparative genome analyses suggest that genetic recombination contributes significantly to genome variations in Pst and may be more important than expected for the origin of globally dispersed isolates. Consistent with this inference, high levels of genetic diversity were observed in Pst populations from western China and central Asia [7] , [46] , where susceptible Berberis species are widely distributed [9] . Therefore, the role of sexual reproduction in genetic diversity and global epidemics of Pst should be considered important and further assessed by sequencing additional Pst isolates and performing population-level comparative analyses. Strains and DNA preparation A single-spore isolate of Pst- CY32 (ref. 15 ) was reproduced on seedlings of wheat cultivar Mingxian169. Five additional Pst strains isolated from Shaanxi province of China, USA, Pakistan, Hungary, and Australia were assayed for their virulence on 17 international differential wheat cultivars [45] , [47] and used for re-sequencing. Urediniospores were harvested and used for DNA isolation by the CTAB/SDS method. High molecular weight genomic DNA was isolated with the Gentra Puregene Cell Kit (Qiagen) and separated on a 1% agarose gel with a Bio-Rad CHEF-DR II electrophoresis apparatus. The 35–45 kb DNA fraction was isolated from the CHEF gel and used for fosmid library construction [48] . Genome sequencing and gene prediction The dikaryotic Pst -CY32 strain was sequenced by Illumina GA and assembled by a ‘fosmid-to-fosmid’ strategy using SOAP denovo [16] , [17] and Celera Assembler [18] ( Supplementary Fig. S1 ). The protein-coding genes were predicted with a combination of homology-based prediction (Genewise (wise2-2-0), GeneMark-ES (version 2.3a), Augustus (version 2.5) and EST-based prediction. The resulting predictions were integrated using Glean (glean-1-0-1) [49] , [50] . The integrated gene collection was searched against the TE database to remove TE-related fragments, and genes encoding peptides shorter than 50 amino acids were filtered out ( Supplementary Data 9 ). Reciprocal blast analysis of Pst , Pgt and Mlp coding sequences was conducted with BlastP V2.2.23 (e-value 1e−7). Hcluster_sg V0.5.0 was used for gene family clustering [51] , [52] . Solar V0.6.9 was used to remove redundant members (Match rate ≥0.33) [20] . TEs and tandem repeats were identified by de novo and knowledge based (Repbase Update, v. 17.11) strategies for all three rust fungi with REPET [53] ( http://urgi.versailles.inra.fr/index.php/urgi/Tools/REPET ). SNV detection To assess the heterozygosity rate and its distribution, high-quality reads (average quality score of >20) from WGS sequencing of three short-insert libraries (224-bp inserts, total clean reads of 3,322 Mb) were realigned to the reference assembly with SOAPaligner (version 2.21) [23] . The probabilities of every possible genotype for each position on the reference genome were calculated, and a statistical model based on Bayesian theory and the Illumina quality system was used to call SNVs. The allelic sequence with the highest probability was used as the reference sequence, and heterozygous SNVs were called if other alleles also had high probability [23] , [54] . Secretome and subcellular targeting prediction SPs of Pst , Pgt , Mlp , Um , Fg , Lb and Bg were identified by the same methodology [12] . SignalP3.0 was used to predict signal peptides. Tmhmm-2.0c and Targetp-1.1 were used to predict proteins with transmembrane domains and targeting to mitochondria, respectively. GPI (glycosylphosphatidyl inositol)—anchor proteins were identified with big-PI FungalPredictor [26] , [27] , [28] . Re-sequencing and genetic variation analysis PE (paired ends) libraries with 500-bp inserts for every Pst isolate were sequenced using Illumina technology by WGS strategy. High-quality reads were compared with the reference sequence of Pst -CY32 by SOAPaligner (SOAP_snp and SOAP_InDel) to identify highly confident SNPs and InDels. Phylogenic trees of Pst isolates based on total SNPs and cSNPs were constructed with TreeBeST-1.9.2 (PHYML) and NJ (bootstraps: 100). Virulence clustering of the seven Pst isolates was done using Heatmap.2. Accession codes: Sequence data for Puccinia striiformis f. sp. tritici CY32 have been deposited in Genbank nucleotide database under accession code ANHQ00000000 . How to cite this article: Zheng, W. et al . High genome heterozygosity and endemic genetic recombination in the wheat stripe rust fungus. Nat. Commun. 4:2673 doi: 10.1038/ncomms3673 (2013).